High-throughput and quantitative assessment of enhancer activity in mammals by CapStarr-seq Cell-type specific regulation of gene expression requires the activation of promoters by distal genomic elements defined as enhancers. The identification and the characterization of enhancers are challenging in mammals due to their genome complexity. Here we develop CapStarr-Seq, a novel high-throughput strategy to quantitatively assess enhancer activity in mammals. This approach couples capture of regions of interest to previously developed Starr-seq technique. Extensive assessment of CapStarr-seq demonstrates accurate quantification of enhancer activity. Furthermore, we find that enhancer strength is associated with binding complexity of tissue-specific transcription factors and super-enhancers, while additive enhancer activity isolates key genes involved in cell identity and function. The CapStarr-Seq thus provides a fast and cost-effective approach to assess the activity of potential enhancers for a given cell type and will be helpful in decrypting transcription regulation mechanisms. Recent advances in epigenomics have enabled genome-wide identification of enhancers in various tissues and species [1] . However, these do not allow direct quantification of enhancer activity. Besides, previous studies have focused their efforts on the isolation of enhancers using high-throughput gene reporter assays coupled to cell sorting [2] , [3] or tags sequencing [4] , providing limited quantitative information. Recently, a technique named Starr-seq enabling genome-wide quantification of enhancer activity in Drosophila cell lines has been developed [5] , [6] , [7] . Although Starr-seq was also applied to human cells using selected BACs [5] , one major limitation for its implementation to mammalian systems resides in their genome size and complexity, rendering challenging the preparation of representative libraries and requiring very high sequencing depth. To circumvent this problem, we have developed CapStarr-seq, a technique capturing genomic sequences of interest for high-throughput assessment of enhancer activity in mammals. We demonstrate the accuracy of the approach to quantify enhancer activity and its efficiency to identify known enhancers in a murine T-cell model. Furthermore, we show that enhancer activity assessed by CapStarr-seq is linked to the epigenetic environment, the transcription factors complexity and the genomic conservation. Finally, we illustrate the interest of CapStarr-seq to study gene regulation of complex loci. CapStarr-Seq is applicable to a wide range of biological questions and will provide an efficient tool to better decipher mechanisms involved in gene regulation. Experimental design of the CapStarr-seq approach To define cis -regulatory modules (CRMs) in developing mouse thymocytes, we analysed DNaseI-seq along with ChIP-seq for ETS1, GATA3, HEB (TCF12), Ikaros, RUNX1 and TCF1 lymphoid-specific transcription factors (TFs) obtained from purified CD4+CD8+ (double positives, DP) thymic population, using a combination of published and newly generated data (see Methods section and Supplementary Tables 1 and 2 ). We identified a set of 7,542 putative CRMs based on the overlap between DNaseI hypersensitive sites (DHS) and regions bound by at least one of the six TFs (average size of the CRMs was 188 bp). To test the enhancer activity of these CRMs we developed CapStarr-seq, a novel approach coupling capture of defined regions to the previously developed Starr-seq technique [5] ( Fig. 1a ; see also Methods section). As a negative control, we included 69 DHS bound by the insulator factor CTCF, which represent open chromatin regions not expected to display enhancer function. In brief, DNA fragments of ∼ 400 bp were captured on a custom-designed microarray covering the complete list of CRMs and cloned by homologous recombination into the mammalian Starr-seq vector [5] . The CapStarr-seq library was transfected into the mouse T-cell line P5424 or the fibroblast cell line 3T3, used as a non-lymphoid control. The P5424 cell line is originated from early developing T cells and resembles DP thymocytes at phenotypic and transcriptomic levels (ref. 8 and Supplementary Fig. 1a,b ). Analyses of GFP expression by FACS demonstrated global enhancer activity of inserted CRMs ( Supplementary Fig. 1c ). Finally, targeted RNA-seq was performed on an Ion PGM sequencer allowing rapid assessment of enhancer activity. As controls, we sequenced the cloned CRM libraries obtained before (hereafter, input) and after transfection. We observed a high recovery of captured CRMs in the input sample (median coverage of 76 FPKM; Supplementary Fig. 1d ) and no bias due to transfection ( Supplementary Fig. 1e ). Moreover, the two CapStarr-seq replicates performed in P5424 cells were highly correlated ( R 2 =0.90; Supplementary Fig. 1f ), indicating high reproducibility of the assay. 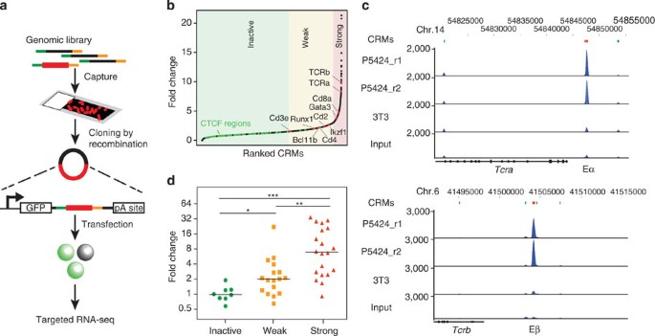Figure 1: Design and experimental validation of the CapStarr-seq approach. (a) CapStarr-seq experimental scheme (see Methods for details). (b) CRMs were ranked in function of their CapStarr-seq fold change (FC) in P5424 cells. CRM activity was defined as follows: inactive (FC<1.5), weak (1.5≤FC<3) and strong (FC≥3). Inactive, weak and strong CRMs are highlighted by green, orange and red background, respectively. Known and characterized T-cell enhancers are plotted in red and were all identified as active CRMs. The CapStarr-seq profiles of these CRMs are shown in Figure 1c andSupplementary Fig. 2. CTCF-bound CRMs are indicated in green. (c) CapStarr-seq profiles highlighting theTcra(Eα; top panel) andTcrb(Eβ; bottom panel) enhancers, which are two strong T-cell enhancers. Each track represents the normalized signal of the CapStarr-seq in the P5424 cell line (two replicates are shown), the 3T3 cell line or the input (captured library). Classification of the CRM activity is indicated by coloured rectangles (green: inactive; orange: weak; red: strong). Mouse genomic coordinates and RefSeq genes are indicated in the top and bottom of each panel, respectively. (d) Enhancer activity of 45 CRMs (8 inactive, 17 weak and 20 strong) was assessed by luciferase reporter assay in triplicate. Values are expressed as the mean fold increase in luciferase counts over the pGL3-promoter vector and normalized by the Renilla intensities (detailed results are presented in theSupplementary Table 3).Y-axis is in Log2 scale. ThePvalues are indicated as follows: *P<0.05; **P<0.01; ***P<0.001 (Student’st-test). Figure 1: Design and experimental validation of the CapStarr-seq approach. ( a ) CapStarr-seq experimental scheme (see Methods for details). ( b ) CRMs were ranked in function of their CapStarr-seq fold change (FC) in P5424 cells. CRM activity was defined as follows: inactive (FC<1.5), weak (1.5≤FC<3) and strong (FC≥3). Inactive, weak and strong CRMs are highlighted by green, orange and red background, respectively. Known and characterized T-cell enhancers are plotted in red and were all identified as active CRMs. The CapStarr-seq profiles of these CRMs are shown in Figure 1c and Supplementary Fig. 2 . CTCF-bound CRMs are indicated in green. ( c ) CapStarr-seq profiles highlighting the Tcra (Eα; top panel) and Tcrb (Eβ; bottom panel) enhancers, which are two strong T-cell enhancers. Each track represents the normalized signal of the CapStarr-seq in the P5424 cell line (two replicates are shown), the 3T3 cell line or the input (captured library). Classification of the CRM activity is indicated by coloured rectangles (green: inactive; orange: weak; red: strong). Mouse genomic coordinates and RefSeq genes are indicated in the top and bottom of each panel, respectively. ( d ) Enhancer activity of 45 CRMs (8 inactive, 17 weak and 20 strong) was assessed by luciferase reporter assay in triplicate. Values are expressed as the mean fold increase in luciferase counts over the pGL3-promoter vector and normalized by the Renilla intensities (detailed results are presented in the Supplementary Table 3 ). 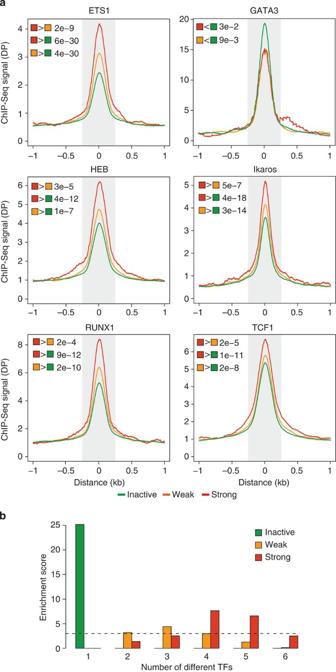Figure 3: Assessment of CRM activity in function of TF binding. (a) Average binding profiles of indicated TFs in DP thymocytes for the inactive, weak and strong CRMs defined in P5424 cells. Statistically significant differences calculated on the regions highlighted in grey are indicated (P<0.05; Mann–WhitneyU-test). (b) Enrichment of the inactive, weak and strong CRM sets in function of the number of different TFs bound. The enrichment score was calculated as the inverted Log10 of thePvalues obtained with a hypergeometric test. Statistically significant enrichments (P<0.001) are indicated by a dotted line. Y -axis is in Log2 scale. The P values are indicated as follows: * P <0.05; ** P <0.01; *** P <0.001 (Student’s t -test). Full size image CapStarr-Seq accurately assesses enhancer activity To define the enhancer activity of each region, we calculated the fold change (FC) of CapStarr-seq over the input signals for each CRM. We then defined three groups of CRMs based on their FC values: inactive (FC<1.5), weak (1.5≤FC<3) and strong (FC≥3) ( Fig. 1b and Supplementary Data 1 ). Strikingly, all the enhancers known to be active in developing T cells displayed either weak or strong CapStarr-seq activity in P5424, but not in 3T3 cells ( Fig. 1b and Supplementary Fig. 2 ). Notably, the Tcra (Eα) and Tcrb (Eβ) enhancers, representing the archetypes of strong T-cell enhancers [9] , were found within the top active CRMs in P5424 cells ( Fig. 1b,c ). In contrast, a CRM close to the ubiquitously expressed Actb gene was active in both cell lines ( Supplementary Fig. 2 ), while 91% of DHS bound by the insulator factor CTCF were found inactive by CapStarr-seq ( Fig. 1b and Supplementary Data 2 ). Thus, the CapStarr-seq approach recapitulates the activity of known T-cell enhancers. To independently confirm the accuracy of CapStarr-seq to identify active enhancers and to discriminate between weak and strong enhancer activity, we tested 45 CRMs in a classical luciferase reporter assay ( Fig. 1d and Supplementary Data 3 ). Of 37 CRMs called active by the CapStarr-seq, 31 displayed significant enhancer activity in the luciferase assay (Student t -test; P <0.01; 12 out of 17 weak and 19 out of 20 strong CRMs). On the contrary, only one of the eight inactive CRMs had significant enhancer activity. Furthermore, the set of strong CRMs demonstrated a statistically higher enhancer activity in the luciferase assay as compared with the weak CRMs (Welch t -test; P =0.0032). Thus, consistency between the two independent reporter assays indicates that high-throughput assessment of enhancer activity by CapStarr-seq is highly accurate and quantitative. CRM activity reflects epigenetic status of endogenous loci To explore whether CapStarr-Seq results reflect the epigenetic status of endogenous enhancers, we analysed ChIP-seq data from the P5424 cell line for H3K4me1, H3K4me2 and RNA-Polymerase II (Pol II), three features generally correlated with enhancer activity [10] . Strong CRMs displayed the highest level of Pol II and H3K4 methylations, while weak CRMs displayed intermediate levels, indicating a positive and quantitative relationship between the CapStarr-seq signal and active epigenetic features ( Supplementary Fig. 3a ). Similarly, the activity of CRMs defined in P5424 cells, but not the one defined in 3T3 cells, was associated with higher levels of Pol II, H3K4me1 and H3K27ac in primary DP thymocytes ( Fig. 2a ). For H3K27ac, which is specifically associated with active enhancers [10] , the differences between the three CRM sets were highly significant when comparing the P5424 selection, but not the 3T3 selection. We and others have previously shown that active enhancers are specifically enriched in H3K4me3 (refs 11 , 12 , 13 ). As high levels of H3K4me3 are generally found in the vicinity of transcription start sites (TSS) [14] , we analysed H3K4me3 enrichments at CRMs distal from any TSS ( Supplementary Fig. 4b ). We found that P5424-defined active CRMs were significantly associated with higher levels of H3K4me3 in both P5424 and DP cells, thus further supporting the link between H3K4 trimethylation and active enhancers. Besides, inactive CRMs were significantly associated with higher levels of the repressive epigenetic mark H3K9me3 and nucleosome occupancy assessed by MNase-seq ( Supplementary Fig. 4a ; note that no consistent differences were observed with H3K27me3), suggesting that inactive CRMs are often in a more closed chromatin configuration and epigenetically silenced, consistent with previous finding [15] . To correlate the activity of the CRMs with gene expression we associated each CRM to the surrounding genes using the GREAT tool [16] . Although genes might be skipped by enhancers [17] , we found that active enhancers in P5424 cells were associated with genes expressed at significantly higher levels in both P5424 cells and DP thymocytes ( Supplementary Fig. 3b and Fig. 2b ). Furthermore, genes associated with strong enhancers displayed significant up- and downregulated expression centred at the DP stages ( Fig. 2c ). 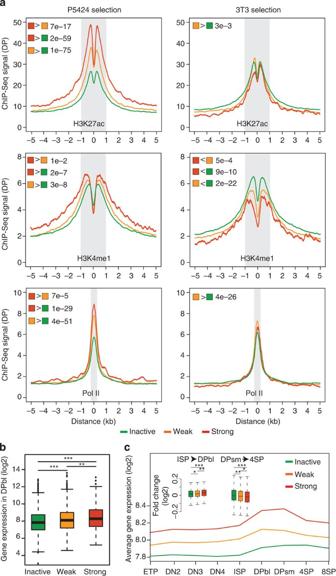Thus, CRM activity assessed by CapStarr-seq reflects epigenetic and transcriptomic status of endogenous loci demonstrating that this approach provides quantitative and qualitative information about enhancer activity in mammals. Figure 2: CapStarr-seq reflects epigenetic status of endogenous enhancers. (a) Average profiles of H3K27ac, H3K4me1 and Pol II ChIP-seq in the mouse DP thymocytes for CRMs identified by CapStarr-Seq as inactive, weak or strong in P5424 (left panels) or in 3T3 (right panels). Statistically significant differences (P<0.05) calculated on the regions highlighted in grey are indicated (Mann–WhitneyU-test). (b) Boxplot showing the expression distribution in primary thymocytes (DPbl: DP blasts) of genes associated with inactive, weak and strong CRMs defined in P5424 cells. (c) Expression dynamic during T-cell differentiation of genes associated with inactive, weak and strong CRMs defined in P5424 cells. Cell populations are as defined by the Immunological Genome Project37and are ordered from less to most differentiated stages. DPbl=double-positive blast; DPsm=double-positive small; DN2-4=double-negative 2–4; ETP=early thymic progenitors; ISP=immature single positive; 4SP and 8SP=single-positive cd4 and cd8, respectively. The inset shows the differential expression between the ISP to DPbl and DPsm to 4SP transitions. In panelsbandc, thePvalues are indicated as follows: *P<0.05; **P<0.01; ***P<0.001 (Student’st-test). Figure 2: CapStarr-seq reflects epigenetic status of endogenous enhancers. ( a ) Average profiles of H3K27ac, H3K4me1 and Pol II ChIP-seq in the mouse DP thymocytes for CRMs identified by CapStarr-Seq as inactive, weak or strong in P5424 (left panels) or in 3T3 (right panels). Statistically significant differences ( P <0.05) calculated on the regions highlighted in grey are indicated (Mann–Whitney U -test). ( b ) Boxplot showing the expression distribution in primary thymocytes (DPbl: DP blasts) of genes associated with inactive, weak and strong CRMs defined in P5424 cells. ( c ) Expression dynamic during T-cell differentiation of genes associated with inactive, weak and strong CRMs defined in P5424 cells. Cell populations are as defined by the Immunological Genome Project [37] and are ordered from less to most differentiated stages. DPbl=double-positive blast; DPsm=double-positive small; DN2-4=double-negative 2–4; ETP=early thymic progenitors; ISP=immature single positive; 4SP and 8SP=single-positive cd4 and cd8, respectively. The inset shows the differential expression between the ISP to DPbl and DPsm to 4SP transitions. In panels b and c , the P values are indicated as follows: * P <0.05; ** P <0.01; *** P <0.001 (Student’s t -test). Full size image CRM activity is linked to TF occupancy and DNA conservation Having validated the CapStarr-seq approach, we asked whether enhancer activity was linked to TF occupancy. First, we quantified the ChIP-Seq signal around the three sets of CRMs for the six TFs initially used to define the CRMs ( Fig. 3a ). Enhancer activity was associated with the strength of ChIP-seq signal for ETS1, HEB, Ikaros, RUNX1 and TCF1. Unexpectedly, the signal for GATA3 was found to be stronger in inactive CRMs as compared with active CRMs, suggesting either a repressive or a pioneering role for this factor. Motif discovery based on the CRM sets identified only the motifs corresponding to the six TFs used in this study ( Supplementary Fig. 5a ; note that ETS1 and Ikaros TFs share the same binding motif [18] ). Moreover, the discovery of GATA motif only in inactive enhancers was consistent with the ChIP-seq results for GATA3. We next asked whether enhancer activity was associated with the complexity of the CRMs by scanning the binding motifs identified for the six TFs by ChIP-seq ( Supplementary Fig. 5b ; overlapping ETS1 and Ikaros sites were count only once). The number of distinct binding sites per CRM was significantly higher in strong CRMs with respect to weak and inactive CRMs ( P =4e−3 and P =3e−4, respectively; Mann–Whitney U -test; Supplementary Fig. 5c ). Similarly, we observed that enhancer activity was associated with the number of TFs bound per CRM ( Fig. 3b ). Indeed, CRMs bound by only one TF were preferentially inactive, while weak and strong CRMs were significantly associated with either 2–4 or 4–5 different TFs, respectively. The reduced enrichment for simultaneous binding of the six TFs in the case of strong CRMs is likely due to the fact that GATA3 is poorly associated with active enhancers. The same tendency was observed when analysing the patterns of enriched CRM sets with respect to the number of distinct TFBS ( Supplementary Fig. 5d ). A striking example is provided by the Ets2 locus where only the CRM bound by five TFs (all except GATA3) displays strong enhancer activity ( Fig. 4a ). Finally, we addressed the question of whether CRM activity was linked to sequence conservation. We computed the phylogenetic conservation among mammalian species for the three sets of CRMs. As shown in Supplementary Fig. 6 , enhancer activity is associated with significantly increased conservation ( P <1e−3; Mann–Whitney U -test), suggesting that highly active enhancers are under strong negative selection [19] . Thus, enhancer activity appears associated with the binding complexity of tissue-specific TFs and sequence conservation. Figure 3: Assessment of CRM activity in function of TF binding. ( a ) Average binding profiles of indicated TFs in DP thymocytes for the inactive, weak and strong CRMs defined in P5424 cells. Statistically significant differences calculated on the regions highlighted in grey are indicated ( P <0.05; Mann–Whitney U -test). ( b ) Enrichment of the inactive, weak and strong CRM sets in function of the number of different TFs bound. The enrichment score was calculated as the inverted Log10 of the P values obtained with a hypergeometric test. Statistically significant enrichments ( P <0.001) are indicated by a dotted line. 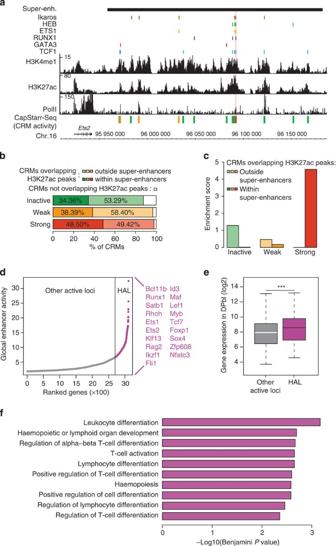Figure 4: Assessment of CRM activity in complex loci. (a) Epigenomic profiles of theEts2locus showing ChIP-Seq signals for H3K4me1, H3K27ac and Pol II in DP thymocytes. Super-enhancers, peaks of the indicated TFs and CRM activities (green: inactive; orange: weak; red: strong) as defined by CapStarr-seq in P5424 cells are also shown. A strong CRM associated with five TFs is highlighted. (b) Distribution of inactive, weak and strong CRMs in function of the overlap with H3K27ac peaks within super-enhancers or outside super-enhancers in DP thymocytes. (c) Enrichment of inactive, weak and strong sets of CRMs overlapping H3K27ac peaks within super-enhancers or outside super-enhancers. The enrichment score was calculated as the inverted Log10 of thePvalues obtained with a hypergeometric test for each CRM set. (d) Genes associated with at least one active CRM were ranked in function of their global enhancer activity in P5424 cells (See Methods). Highly active loci (HAL) were defined as the genes from which the global enhancer activity is beyond the inflexion point. HAL encoding for TFs involved in early T-cell differentiation are listed. (e) Boxplot showing the distribution of gene expression in DPbl thymocytes of HAL and remaining loci (Other active loci) defined in (d). Thick line represents the median expression, and the bottom and top whiskers indicate, respectively, the minimum and the maximum expression level. Statistical significance was calculated by a Student’st-test (P=5e−8). (f) Top 10 of significant gene ontology (GO) terms for biological process found with the list of HAL defined in (d). No significant enrichment was found for the remaining loci (other active loci). Full size image Figure 4: Assessment of CRM activity in complex loci. ( a ) Epigenomic profiles of the Ets2 locus showing ChIP-Seq signals for H3K4me1, H3K27ac and Pol II in DP thymocytes. Super-enhancers, peaks of the indicated TFs and CRM activities (green: inactive; orange: weak; red: strong) as defined by CapStarr-seq in P5424 cells are also shown. A strong CRM associated with five TFs is highlighted. ( b ) Distribution of inactive, weak and strong CRMs in function of the overlap with H3K27ac peaks within super-enhancers or outside super-enhancers in DP thymocytes. ( c ) Enrichment of inactive, weak and strong sets of CRMs overlapping H3K27ac peaks within super-enhancers or outside super-enhancers. The enrichment score was calculated as the inverted Log10 of the P values obtained with a hypergeometric test for each CRM set. ( d ) Genes associated with at least one active CRM were ranked in function of their global enhancer activity in P5424 cells (See Methods). Highly active loci (HAL) were defined as the genes from which the global enhancer activity is beyond the inflexion point. HAL encoding for TFs involved in early T-cell differentiation are listed. ( e ) Boxplot showing the distribution of gene expression in DPbl thymocytes of HAL and remaining loci (Other active loci) defined in ( d ). Thick line represents the median expression, and the bottom and top whiskers indicate, respectively, the minimum and the maximum expression level. Statistical significance was calculated by a Student’s t -test ( P =5e−8). ( f ) Top 10 of significant gene ontology (GO) terms for biological process found with the list of HAL defined in ( d ). No significant enrichment was found for the remaining loci (other active loci). Full size image Super-enhancers are enriched in strong enhancers Super-enhancers were recently defined as a class of cis -regulatory elements spanning large genomic regions associated with clusters of individual DHS and high levels of epigenetic marks, such as H3K27ac [20] , [21] . Super-enhancers were proposed to be more specifically enriched in active enhancers [21] . To address this issue in a high-throughput manner, we defined super-enhancers in DP thymocytes based on H3K27ac signal, using ROSE tool as previously described [20] , [21] . We found that the proportion of CRMs overlapping H3K27ac peaks within super-enhancers increases in function of CRM activity. Indeed, they represent 34, 38 and 48% of the inactive, weak and strong CRMs, respectively ( Fig. 4b ). Remarkably, CRMs overlapping H3K27ac peaks within super-enhancers were significantly and specifically enriched in strong enhancers as compared with those overlapping H3K27ac peaks outside super-enhancers ( Fig. 4c ). Hence, while super-enhancers overlap many inactive CRMs (for example., Ets2 locus, Fig. 4a ; Ikzf1 and Runx1 loci, Supplementary Fig. 7 ), they have a higher probability of containing strong enhancers. Additive enhancer activity reveals cell identity genes Tissue-specific gene regulation is thought to be achieved by the combinatorial effect of multiple enhancers [22] . Hence, we asked whether analysis of additive enhancer strength could provide functional information concerning the regulated genes. We selected genes associated with at least one active CRM and computed the sum of CapStarr-seq FC of their active CRMs to obtain a global enhancer activity for each of these loci (see Methods). Genes ranking in function of the global enhancer activity reveals the existence of 375 loci displaying substantially higher global enhancer activity ( Fig. 4d and Supplementary Data 4 ). These highly active loci (hereafter, HAL) were expressed at significantly higher levels in DP thymocytes as compared with other active loci ( Fig. 4e ) and were exclusively involved in T-cell-related functions ( Fig. 4f ). Note that the set of ‘other active loci’ was not significantly enriched in any biological process. Remarkably, the set of HAL included most of the known regulators of T-cell differentiation and function ( Fig. 4d ), namely Bcl11b , Runx1 , Ets1 , Ikzf1 , Lef1 , Myb and Tcf7 , which encode crucial TFs involved in early T-cell differentiation [23] . Moreover, HAL were often associated with several weak and strong CRMs (for example, Ets2 locus, Fig. 4a ; Ikzf1 and Runx1 loci, Supplementary Fig. 7 ). This suggests that key genes involved in cell identity are regulated by additive enhancer activities, likely allowing integration of different environmental inputs and conferring higher transcriptional output. We developed a CapStarr-seq approach coupling capture of defined genomic regions to the previously developed Starr-seq technique. Our method takes advantage of targeted enrichment of CRMs of interest as well as rapid sequencing with an Ion PGM technology, providing a fast and cost-effective approach for the study of enhancer activity in mammals. As an initial assessment of the CapStarr-seq technique, we analysed here a set of 7,542 CRMs overlapping DHS bound by at least one lymphoid TF in primary developing mouse thymocytes. We extensively validated the accuracy of CapStarr-seq to quantify enhancer activity in mammals and demonstrated its robustness to discriminate between weak and strong enhancers. We explored the benefits of this approach on the understanding of molecular basis driving enhancer activity, including epigenetic features and combinatorial binding of TFs. Moreover, we showed that computing additive enhancer activity enables the identification of HAL that overlap genes highly relevant to cell identity. Starr-seq has been efficiently achieved with the full drosophila genome [5] , which represent ∼ 48-fold the set of CRMs analysed in this study and ∼ 7-fold the estimated genome space covered by all potential enhancers in a given mammalian cell type (estimation based on the average number of total DHS per cell type [24] ). It is therefore possible to extend the use of CapStarr-seq to a larger genomic scale, providing that the genomic regions could be captured. This might be achieved by either using higher-density arrays and/or combining multiple arrays. In the future, it is expected that the CapStarr-Seq approach will be applied to explore the activity of all potential enhancers for a given cell type, while including additional negative controls like random or DNaseI-insensitive regions. Together our findings illustrate how the CapStarr-seq technique will further help to the functional assessment of mammalian enhancers that are active in different cellular systems. This approach will be also useful for thorough characterization of enhancer subsets involved in specific pathways or induced by specific stimuli. Mouse and cell culture C57/Bl6 mice were housed under specific pathogen-free conditions and handled in accordance with French and European directives (EU Agreement N° A-13013 03). This work was approved by the Aix-Marseille University Institutional Animal Care and Use Committee. Only male mice were used in this study and were killed for analysis between 4 and 6 weeks of age. DP thymocytes were purified as previously described [25] . P5424 cells [8] (kindly provided by Dr. Eugene Oltz, Washington, USA) and NIH-3T3 (3T3, ATCC: CRL-1658) cells were cultured in RPMI medium (Life technologies) supplemented with 10% heat-inactivated FBS (PAA) at 37 °C. ChIP-seq Chromatin preparation and ChIPs [25] were performed with DP thymocytes and P5424 cell line. In brief, after purification, crosslinked nuclei from DP thymocytes or P5424 cells were sonicated using a Misonix 4000 (Misonix Inc) sonicator for 7 cycles (30 s on, 30 s off, amplitude 40). After the addition of Triton X-100 to a final concentration of 1%, debris was removed through centrifugation at 20,000 g and 4 °C for 20 min. Extracts were incubated overnight at 4 °C on a rotating wheel with antibodies bound to protein G Dynabeads (Life technologies). The anti-TCF1 antibodies used were # 2203 (cell signaling, 20μL); the anti-HEB antibodies used were # sc-357X (Santa cruz, 10 μg); the anti-RNA Polymerase II used were # sc-899x (Santa cruz, 4 μg); the anti-H3K4me1 antibodies used were # ab8895 (Abcam, 1 μg); the anti-H3K4me2 used were # ab32356 (Abcam, 1 μg); the anti-H3K4me3 used were # ab8580 (Abcam, 1 μg); the anti-H3K9me3 used were # ab8898 (Abcam, 2 μg) and the anti-H3K27ac used were # ab4729 (Abcam, 2 μg). Beads were washed five times in RIPA buffer (50 mM Hepes pH 7.6, 500 mM LiCl, 1 mM EDTA pH 8, 1% NP-40, 0.7% Na-Deoxycholate), once in TE+ (10 mM Tris pH 8, 1 mM EDTA pH 8, 50 mM NaCl) and once in TE (10 mM Tris pH 8, 1 mM EDTA pH 8). Immunoprecipitated chromatin was recovered from the beads with two subsequent elution steps at 65 °C for 15 and 10 min in elution buffer (NaHCO3 100 mM, 1% SDS). The two eluates were combined and incubated at 65 °C overnight (13–15 h) for crosslink reversal in the presence of proteinase K. DNA was purified using QIAquick PCR purification kit (Qiagen). At least 1 ng of ChIP was used for library preparation. Libraries for the TCF1 and HEB ChIPs in DP thymocytes were prepared according to the SOLiD ChIP-Seq protocol and sequenced on 5500 SOLiD System (Life technologies), according to the manufacturer’s instructions. Libraries for ChIPs against H3K4me1, H3K4me2, H3K4me3, H3K9me3, H3K27ac and Pol II were prepared according to Illumina ChIP-Seq protocol and sequenced on a HighSeq 2000 (Illumina) according to the manufacturer’s instructions. DNaseI-seq DNase I digestion [26] and high-throughput sequencing were performed on intact nuclei from DP thymocytes. In brief, nuclei were extracted using NP-40 in an isotonic buffer. The NP-40 detergent was removed and the nuclei were incubated for 3 min at 37 °C with limiting concentrations of the DNA endonuclease, DNase I (Sigma-Aldrich) supplemented with Ca 2+ and Mg 2+ . The digestion was stopped with EDTA and the samples were treated with proteinase K. The small double-hit fragments (<500 bp) were recovered by high-resolution agarose gel electrophoresis followed by gel purification. DNase I hypersensitive sites were sequenced on a 5500 SOLiD System. ChIP-seq and DNaseI-seq data processing ChIP-seq data sets for Pol II, MNase, the transcription factors (TFs) ETS1, GATA3, Ikaros, RUNX1 and CTCF in DP thymocytes were downloaded from Gene Expression Omnibus (GEO) database ( Supplementary Table 2 ). ChIP-seq for all TFs and DNaseI-seq samples were mapped to the mouse genome (assembly NCBI37/mm9) using BFast tool (v0.7.0) [27] and only reads that have a unique best scoring alignment were used. ChIP-seq for Pol II, H3K4me1, H3K4me2 and H3K4me3 in P5424 cell line was mapped to the mouse genome (assembly NCBI37/mm9) using the Illumina’s integrated Eland software. To exclude redundancies from PCR amplification, we counted only unique fragments. Fragment size was computed using the Hypergeometric Optimization of Motif EnRichment (HOMER) tool (v6.1) [28] ( Supplementary Table 1 ). Read-count intensity profiles (wiggle files) were constructed by elongating each mapped read to the estimated fragment size, and counting the elongated read overlaps within a window of 50 nucleotides after normalization of the profile by the number of mapped reads. Peak-calling was performed using the HOMER tool with default settings (FDR: 0.001; local and input fold enrichment: 4.0).. Processed data for Pol II, MNase and epigenetic modifications H3K4me1, H3K4me3, H3K27ac and H3K27me3 in DP thymocytes were downloaded from GEO [25] , [29] , [30] . ChIP-seq data were visualized using the Integrated Genome Browser ( http://bioviz.org/igb/ ). Identification of CRMs CRMs were extracted by merging peaks of TFs ETS1, GATA3, HEB, Ikaros, RUNX1 and TCF1 that overlap DNaseI peaks. These resulted in a set of 7,542 CRMs that were retained to design the capture microarray ( Supplementary Data 1 ; the average size of the CRMs was 188 bp). As a control, we included 69 CTCF peaks ( Supplementary Data 2 ). Generation of genomic library for CapStarr-seq Genomic DNA from C57bl6 mouse thymus was sheared by sonication (Diagenode pico), and DNA fragments between 330 and 430 bp were size-selected on a 1.2% high-resolution agarose gel (Sigma-Aldrich) and purified using Qiaquick gel extraction kit (Qiagen). Size-selected genomic DNA was analysed by Bioanalyzer (Agilent) and the average size estimated at 400 bp. Ion Torrent adapters were ligated to 8 μg of size-selected DNA fragments using Ion Plus Fragment Library Kit (Life Technologies) following the manufacturer’s instructions except for the final PCR amplification. Forty individual PCR reactions (98 °C for 2 min; followed by 10 cycles of 98 °C for 20 s, 65 °C for 15 s, 72 °C for 15 s) with 2 μl of adaptor ligated DNA were performed using KAPA Hifi Hot Start Ready Mix (KAPA Biosystems) and primers (fw: 5′-TAGAGCATGCACCGGAACCATCTCATCCCTG*C*G*T*G-3′ and rw: 5′-GGCCGAATTCGTCGAAACCACTACGCCTCCGC*T*T*T*C-3′; * indicates phosphorothioate bonds) that add a specific 15 nucleotides extension for directional cloning by homologous recombination (In Fusion HD, Clontech). PCR reactions were pooled and purified with Agencourt AMPureXP DNA beads (Ratio beads/PCR 1.2; Beckman Coulter). Capture of genomic library For target enrichment, a home-designed 3 bp resolution oligonucleotide microarray covering the 7,542 CRMs defined in section 5 was constructed using the SureSelect technology (Agilent) and the eArray tool default setting ( https://earray.chem.agilent.com/earray/ ). The genomic library was hybridized on the microarray as outlined in the Agilent SureSelect DNA Capture Array protocol (Agilent). In brief, 10 μg of PCR (in 138 μl), 5 μl Blocking oligo 1 5′-(TAGAGCATGCACCGGAACCATCTCATCCCTG*C*G*T*G)-3′ (200 μM), 5 μl Blocking oligo 2 5′-(GGCCGAATTCGTCGAAACCACTACGCCTCCGC*T*T*T*C)-3′ (200 μM), 5 μl Blocking oligo 3 5′-(CACGCAGGGATGAGATGGTTCCGGTGCATGC*T*C*T*A)-3′ (200 μM), 5 μl Blocking oligo 4 5′-(GAAAGCGGAGGCGTAGTGGTTTCGACGAATTC*G*G*C*C)-3′ (200 μM), 50 μl Mouse Cot-1 DNA (1 mg ml −1 ), 52 μl 10 × blocking buffer and 260 μl 2 × Hyb buffer were mixed and denatured at 95 °C for 3 min followed by transfer to 37 °C for 30 min. The mixture was centrifugated at 17,800 g for 1 min. Four hundred and ninety microlitres of hybridization mixture was dispensed onto the centre of a gasket slide in the hybridization chamber. The oligonucleotide array was placed with the active side contacting the hybridization mixture. The resulting slide-gasket sandwich was incubated at 65 °C for 65 h on a rotisserie in an Agilent hybridization oven. The aCGH Wash buffer 2 was preheated at 37 °C in a hybridization oven overnight before washing. Following hybridization, the slide-gasket sandwich was disassembled in aCGH wash buffer 1 at room temperature. The slide was washed for 10 min in wash buffer 1 and transferred to wash buffer 2 at 37 °C and washed for 5 min. Slides were dried and 490 μl of nuclease-free water were added to a new gasket slide and the dried μarray was placed atop as described earlier, creating a fresh slide-gasket sandwich. The slide-gasket sandwich was incubated at 95 °C for 10 min on a rotisserie in an Agilent hybridization oven. After heat denaturation, the eluate was recovered with a 1-ml 30G syringe. The eluted DNA was purified with Agencourt AMPureXP DNA beads (Ratio beads/PCR 1.8) and eluted in 80 μl. Twenty independent 25 μl PCR (98 °C for 2 min; followed by 20 cycles of 98 °C for 20 s, 65 °C for 15 s, 72 °C for 15 s) reactions with 4 μl of captured DNA were performed using KAPA Hifi Hot Start Ready Mix and primers (fw: 5′-TAGAGCATGCACCGGAACCATCTCATCCCTG*C*G*T*G-3′ and rw: 5′-GGCCGAATTCGTCGAAACCACTACGCCTCCGC*T*T*T*C-3′). PCR reactions were pooled, purified with Agencourt AMPureXP DNA beads (Ratio beads/PCR 1.8) and eluted in 200 μl H 2 O. Library cloning The mammalian STARR-Seq screening vector [5] has been kindly provided by Alexander Stark (Vienna, Austria). The screening vector was linearized by a 6 h digestion with AgeI-HF and SalI-HF (New England Biolabs), followed by agarose gel electrophoresis, QIAquick gel extraction (Qiagen) and a clean-up with Qiagen Minelute PCR purification Kit (Qiagen). A total of 500 ng of amplified captured DNA were recombined (Clontech In-Fusion HD) with 500 ng of the linearized screening vector (Qiagen) in a total of ten 10-μl reactions (each containing 50 ng of captured DNA and 50 ng of screening vector). The recombination reactions were pooled, purified with Agencourt AMPureXP DNA beads and eluted in 29 μl. Thirteen aliquots (20 μl each) of MegaX DH10B Electrocompetent Bacteria (Life technologies) were transformed with 2 μl of DNA each, according to the manufacturer’s recommendation. After 1 h recovery at 37 °C, transformations were pooled and transferred to 2 l of LB AMP medium and grown overnight. Aliquots of the transformation were plated on LB AMP to estimate the number of cloned fragments. Finally, the plasmid library was extracted using Qiagen Plasmid Plus Mega Kit (Qiagen). Library transfection Transfection of library (5 μg/1 × 10 6 cells) was performed using Neon Transfection System (Life technologies). A total of 30 × 10 6 cells were transfected per experiment. A total of 25 × 10 6 cells were used for RNA purification and 5 × 10 6 for DNA purification. P5424 cells were transfected with 1600v-20ms-1 pulse and 3T3 with 1400v-20ms-2 pulses. Transfected cells were transferred to complete growth medium and incubated for 24 h before RNA and DNA isolation. RNA and plasmid isolation from transfected cells Total RNA was extracted using RNeasy miniprep kit (Qiagen) with the on-column DNaseI treatment. The PolyA RNA fraction was isolated using μMACS mRNA isolation kit (Milteny) following the manufacturer’s instructions. PolyA RNA was treated with Ambion turboDNase (Ambion) and purified with RNeasy Minelute kit (Qiagen). Finally, mRNA was quantified with Qubit RNA HS Kit (Life technologies). Plasmid DNA was extracted from 5 × 10 6 cells using a QIAGEN plasmid plus mini kit (Qiagen), following the manufacturer’s instructions. Reverse transcription and sequencing library preparation First strand cDNA synthesis was performed with superscript III (Life technologies) using a reporter-RNA specific primer (5′-CAAACTCATCAATGTATCTTATCATG-3′) and 0.2 to 0.3 μg of polyA RNA per reaction for a total of 10 reactions. After reverse transcription, 1 μl of RNaseH was added (37 °C, 1 h). The cDNA was purified with QIAquick PCR purification kit and concentration was determined with Qubit ssDNA Kit (Life technologies). The cDNA was amplified by a 2-step nested PCR using the KAPA Hifi Hot Start Ready Mix. In the first PCR (98 °C for 2 min; followed by 15 cycles of 98 °C for 20 s, 65 °C for 20 s, 72 °C for 30 s), 5 ng of cDNA per reaction was amplified using two reporter-specific primers (fw: 5′-GGGCCAGCTGTTGGGGTG*T*C*C*A*C-3′ and rw: 5′-CTTATCATGTCTGCTCGA*A*G*C-3′), one of which spans the splice junction of the synthetic intron, in a total of 10 reactions. To remove any residual contamination of plasmid or cDNA, PCR products were purified on gel using QIAquick gel extraction Kit (Qiagen) followed by a clean-up with QIAquick minelute PCR purification kit (Qiagen). To generate the Ion Torrent libraries, the purified PCR was used as a template for the second PCR (5 ng/PCR, for a total of 10 PCR; 98 °C for 2 min; followed by 10 cycles of 98 °C for 20 s, 65 °C for 20 s, 72 °C for 30 s) with the KAPA Hifi Hot Start Ready Mix and Ion Torrent library amplification primer mix (Life technologies, T_PCR_A: 5′-CCA TCT CAT CCC TGC GTG TC-3′ and P1amp: 5′-CCA CTA CGC CTC CGC TTT CCT CTC TAT G-3′). To generate the INPUT control, 10 reactions with 5 ng of reporter constructs (library) per reaction were amplified using the same conditions as above, at the exception of the forward primer in the first PCR (fw: 5′-GGGCCAGCTGTTGGGGTG*A*G*T*A*C-3′). To assess potential biased in library composition caused by electroporation, 10 reactions with 5 ng per reaction of reporter constructs isolated from transfected cells were amplified as described above. Ion Torrent sequencing The emulsion PCRs were performed with 25 μl of Starr-Seq libraries (10 pM) using the Ion PGM Template OT2 400 kit and the ONE TOUCH 2 system (Life Technologies), according to the manufacturer’s instructions. Template-positive Ion Sphere Particles were enriched using the Ion PGM Enrichment Beads (Life Technologies), according to the manufacturer’s instructions. Finally, libraries were sequenced on ION 318 Chip v2 (Life Technologies) using the Ion PGM Sequencing 200 kit (Life Technologies), according to the manufacturer’s instructions. CapStarr-seq data processing Sequencing data of CapStarr-seq samples were mapped to the mouse genome using the Ion PGM TM pipeline ( Supplementary Table 1 ). Wiggle files were generated as described in section 4. To quantify the coverage of each CRM, we intersected the elongated mapped reads (that is, fragments) with the CRMs using BedTools (v2.17.0) [31] and calculated FPKM values (Fragment Per Kilobase per Million mapped reads). After processing the two P5424 biological replicates separately to assess reproducibility ( R 2 =0.90), we pooled both replicates and re-computed FPKM values for all subsequent analyses. To filter out CRMs not captured by the array, all CRMs with a FPKM lower than 1 in the input sample were excluded, thereby removing 390 CRMs. A total of 7,152 CRMs were then retained for further analyses (genomic coordinates are provided in Supplementary Data 1 ). The enrichment of CapStarr-seq samples over input was computed by calculating the ratio of FPKM. The FC was used to determine the enhancer activity of each CRM. CRMs with a FC lower than 1.5 were labelled ‘inactive’, CRMs with a FC between 1.5 and 3 were labelled ‘weak’ and CRMs with a FC equal or higher than 3 were labelled ‘strong’ ( Supplementary Data 1 ). We identified 4,440 inactive, 2,279 weak and 433 strong CRMs in the P5424 pooled sample, and 4,407 inactive, 2,559 weak and 186 strong CRMs in the 3T3 sample. Of these 1,205 (33%) weak and 75 (24%) strong CRMs were common to the two cell types. CapStarr-seq data were visualized using the UCSC genome browser ( https://genome.ucsc.edu/ ). FACS analysis A total of 5 × 10 6 P5424 cells were transfected, as described above, with the empty STARR-Seq screening vector or the STARR-Seq screening vector containing the library. Twenty-four hours post electroporation, GFP expression was assessed on a FACSCalibur (BD Biosciences). For CD4/CD8 staining, 1 × 10 6 P5424 cells were incubated for 10 min with 5μl of mouse CD4-FITC antibody (Miltenyi, Ref No 130091608) and with 5 μl of Mouse CD8a-PE (Milteny, Ref No 130102595) in 50μL of PBS/0,5% BSA/2 mM EDTA. After washing, CD4 and CD8 expression was analysed on a FACSCalibur (BD Biosciensces). Gene association CRM-associated genes were identified using the online tool GREAT (Genomic Regions Enrichment of Annotations Tool, v2.0.2) [16] with default settings. GREAT assigns each gene a regulatory domain consisting of a basal region of −5 kb/+1 kb from TSS, and an extension up to the nearest gene’s basal region but no more than 1 Mb in both directions. Each CRM is associated with all genes in whose regulatory domains it lies. In all, 73.98% of the CRMs were associated with two genes, 25.94% with only one gene and 0.08% were associated with three genes ( Supplementary Data 1 ). CRMs were defined as ‘distal’ if they were located at more than 2 kb upstream and 1 kb downstream the TSS of any annotated gene. Motif discovery and scanning The RSAT (Regulatory Sequence Analysis Tools) [32] , [33] suite was used to perform a de novo motif analysis (peak-motifs tool) in the different TF ChIP-seq peaks and CRM sets identified in P5424 cells, as well as in the whole set of CRMs ( Supplementary Fig. 5 ). We used the matrices for ETS1/Ikaros, GATA3, HEB, RUNX1 and TCF1 identified by ChIP-seq to scan the three sets of CRMs. To assess the quality of the matrices and to determine thresholds to use for the motif scanning, we used the matrix-quality tool from RSAT [34] . We then performed motif scanning in each set of CRMs with adapted thresholds for each matrix using matrix-scan from the same suite. Average profiles Average profiles were generated by extracting ChIP-seq signal from wiggle files around CRMs centre (+/−5 kb for histone modifications, MNase and Pol II; +/−1 kb for TFs). To test whether the differences between inactive, weak and strong CRM sets were statistically significant, we first extracted the average signal of the top 25% signal of each CRM in a region centred on the CRM (+/−1 kb for histone modifications and MNase; +/−250 bp for TFs and Pol II). A Mann–Whitney U -test was then performed between each pair of CRM sets. Gene expression Gene expression data of αβ T cells were downloaded from the Immunological Genome Project website ( www.immgen.org ). A quantile normalization was then applied on gene expression of stages ETP (Early Thymic Progenitor), DN2 (Double Negative stage 2), DN3, DN4, ISP (Immature Single Positive), DPbl (Double Positive blast), DPsm (Double Positive small) and single-positive CD4+ (4SP) and CD8+ (8SP) thymocytes. Gene expression in P5424 cells was analysed in duplicate using the SurePrint G3 Mouse GE 8x60K microarray platform (Agilent). Statistical significance of differences between inactive, weak and strong CRM sets was calculated using a Student t -test. Conservation analysis The genomic evolutionary rate profiling (GERP) scores were used to assess the level of evolutionary constraint of each nucleotide within and around CRMs. GERP scores, downloaded from the UCSC table browser tool (mm9 assembly), are based on an alignment of 22 mammals to the Mus musculus genome (mm9) and have a maximum level of 4.14. The average profile (+/−1 kb from the CRM centre) was generated by smoothing GERP scores with a window of 50 bp. Statistical significance of differences between inactive, weak and strong CRM sets was calculated by taking into account the average GERP scores in each CRM and applying a Mann–Whitney U -test. Identification of super-enhancers Super-enhancers in DP thymocytes were identified using H3K27ac peaks and ROSE tool ( http://bitbucket.org/young_computation/rose ) [35] with the sequence alignment files of H3K27ac and Input samples, the default stitching distance of peaks (12.5 kb) and an exclusion region of +/−2.5 kb around TSSs to account for promoter biases. We identified 1,044 super-enhancers. H3K27ac peaks falling within super-enhancers were called ‘super-enhancer peaks’ and those falling outside super-enhancers were labelled ‘single peaks’. The overlap of H3K27ac peaks with CRMs was performed using BedTools. The enrichment of CRMs in H3K27ac peaks was calculated using a hypergeometric test. Identification of highly active loci We first summed up the fold changes of active CRMs (weak and strong CRMs) associated with each gene. Genes associated with only inactive CRMs were not included in the analysis. HAL were then determined by identifying an inflection point of the global enhancer activity (sum of fold changes) versus gene rank. The inflection point was computed by determining the diagonal line of the curve from end points, and by sliding this diagonal line to find where it is tangential. We identified 375 HAL ( Supplementary Data 4 ). Enrichments of HAL or remaining loci in gene ontology terms for biological process were calculated using DAVID tool [36] with default settings (count threshold: 2; EASE threshold: 0.1; multiple testing correction by the Benjamini procedure) and the set of genes associated with CRMs as a background model. Reporter assay A total of 1 × 10 6 P5424 cells were transiently transfected in six-well plates with 200 ng of Renilla vector along with 1 μg of pGL3-promoter vector (Promega) or pGL3-promoter vectors containing the specified genomic regions cloned downstream the Luciferase gene ( Supplementary Data 3 ). The transfection was performed with NEON 100 μl transfection kit (Life technologies) according to the manufacturer’s protocol. Twenty-four hours after transfection, cells were washed once with 1 × PBS and the luciferase assay (Dual-Luciferase Reporter Assay System, Promega) was performed according to the manufacturer’s protocols. Values are expressed as fold increase in luciferase counts over the pGL3-promoter vector and normalized by the Renilla intensities. All experiments were performed in triplicates. Accession codes: Sequencing data generated in this study have been submitted to the NCBI Gene Expression Omnibus ( http://www.ncbi.nlm.nih.gov/geo/ ) under the GEO accession numbers GSE60029 , GSE63732 and GSE63416 (details in Supplementary Table 1). Transcriptome data for P5424 cell line are available under the GEO accession number GSE63731 . How to cite this article: Vanhille, L. et al. High-throughput and quantitative assessment of enhancer activity in mammals by CapStarr-seq. Nat. Commun. 6:6905 doi: 10.1038/ncomms7905 (2015).